Contribution of RNA polymerase concentration variation to protein expression noise Cell-to-cell variation in gene expression, or noise, is a general phenomenon observed within cell populations. Transcription is known to be the key stage of gene expression where noise is generated, however, how variation in RNA polymerase (RNAP) concentration contributes to gene expression noise is unclear. Here, we quantitatively investigate how variations in absolute amounts of RNAP molecules affect noise in the expression of two fluorescent protein reporters driven by identical promoters. We find that intrinsic noise is independent of variation in RNAP concentrations, whereas extrinsic noise, which is variation in gene expression due to varying cellular environments, scales linearly with variation in RNAP abundance. Specifically, the propagation of RNAP abundance variation to expressed protein noise is inversely proportional to the concentration of RNAP, which suggests that the change in noise that results from RNAP fluctuations is determined by the fraction of promoters that is not occupied by RNAP. Even a population of genetically identical cells exhibits different levels of protein expression, which is termed cell-to-cell variation or noise [1] , [2] . Noise, an unavoidable phenomenon in biochemical reactions, often shows crucial functional roles in cells, such as resulting in state switching, differentiation and cell fate determination [3] , [4] , [5] , [6] . Typically noise is generated during the two central gene expression processes, that is, transcription by RNA polymerase (RNAP) and translation by the ribosome; these processes are associated with a small number of templates, such as genes and messenger RNAs (mRNAs) [7] , [8] . When protein expression levels are low (<10 copies per cell), intrinsic noise, originating from the innate stochasticity of biochemical reactions [2] , is the dominant source of total noise: intrinsic noise is inversely proportional to the protein expression level [9] . However, as the protein expression level increases, the total noise decreases and reaches a saturation floor, or lower limit, in both bacteria and yeast [9] , [10] , [11] , [12] . This limit is thought to originate mostly from extrinsic noise, that is, the variation in gene expression brought by varying cellular environments that are extrinsic but influence the rate of gene expression, which is a dominant source of total noise when the protein expression level is sufficiently high [1] , [9] , [13] , [14] , [15] . Various factors, such as cellular differences due to the cell cycle [16] , [17] and variation in the concentration of essential cellular proteins, such as RNAP, ribosomal proteins, transcription factors and other metabolites, contribute to extrinsic noise [15] , [18] , [19] , [20] . Indeed, cell cycle differences contribute to extrinsic noise in bacteria, but a substantial amount of extrinsic noise remains following cell cycle correction [16] . Although extrinsic noise is believed to be the major factor determining total noise [1] , how noise sources other than the cell cycle generate and control extrinsic noise has not yet been properly addressed experimentally. For example, how the gene expression machinery proteins, such as RNAP and ribosomal proteins, generate or regulate extrinsic noise has not been investigated, because these proteins are essential factors: variation in their concentrations or distributions significantly alters gene expression profiles. Through the use of different promoter- or ribosome-binding site sequences to vary expression levels, the effects of transcriptional and translational efficiency on noise have been described [7] , [21] . However, these studies did not directly vary the concentration of RNAP. Here, we develop a new gene expression system for measuring noise in RNAP expression together with the noise in the expression of downstream proteins. To control the RNAP expression level so that variations in its expression would have a minor effect on cell growth conditions, we use yellow-fluorescent-protein (YFP)-fused T7 RNAP in Escherichia coli and placed two fluorescent reporter genes, cyan-fluorescent protein (CFP) and mCherry, under the control of identical copies of the T7 RNAP promoter ( Fig. 1a ). Tagging T7 RNAP with YFP allows us to monitor the concentration of T7 RNAP in individual cells. The two fluorescent proteins, CFP and mCherry, are used to measure both intrinsic noise, that is, variations between CFP and mCherry expression levels within the same cell, and extrinsic noise, that is, variations in CFP or mCherry expression levels between cells ( Fig. 1b ) [1] . We observe that RNAP concentration variation indeed propagates to downstream protein expression noise, contributing only to extrinsic noise. The efficiency of the propagation of RNAP noise to downstream protein noise is inversely proportional to the concentration of RNAP. Remarkably, when RNAP noise is diminished, even without correcting for cell cycle heterogeneity and possible variations in the concentrations of other extrinsic noise factors, extrinsic noise is markedly reduced to 30% of the noise limit observed in E. coli proteins [9] . This result suggests that the transcriptional noise caused by RNAP is the major source of the total noise of highly expressed proteins in E. coli . 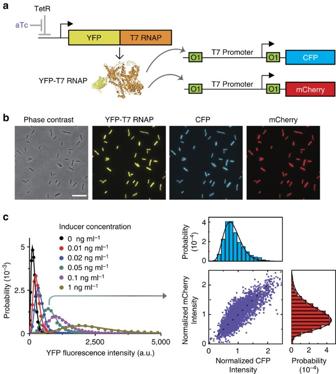Figure 1: Genetic design for achieving T7 RNAP-driven expression of dual fluorescent proteins inE. coli. (a) A schematic description of the T7 RNAP-driven gene expression system. YFP-fused T7 RNAP is expressed from a tetracycline promoter in the pNL001 plasmid. The inducer anhydrotetracycline (aTc), which binds to the tet repressor, controls the expression level of YFP-fused-T7 RNAP. Then, the genes encoding CFP and mCherry, which are integrated intoE. coligenomic DNA, are expressed by T7 RNAP. Two Lac operators (O1) are located upstream and downstream of the T7 promoter. To achieve full expression of CFP and mCherry, 1 mM isopropyl β-D-1-thiogalactopyranoside (IPTG) was added. (b) Representative phase contrast, YFP, CFP and mCherry images ofE. coliNL010 carrying pNL001. Scale bar, 10 μm. (c) Steady-state distributions of YFP-T7 RNAP at different aTc concentrations. Each distribution fits a gamma distribution well (solid curves). (d) Correlation between the CFP and mCherry intensity in the NL010 strain, in which T7 RNAP is induced under an aTc concentration of 0.05 ng ml−1(green curve inFig. 1c). Each point represents a cell, for which fluorescence intensities are normalized by the average intensities of the cell population. The distributions of the CFP (top) and mCherry (right) intensities are described well by the gamma functions (solid curves). Figure 1: Genetic design for achieving T7 RNAP-driven expression of dual fluorescent proteins in E. coli . ( a ) A schematic description of the T7 RNAP-driven gene expression system. YFP-fused T7 RNAP is expressed from a tetracycline promoter in the pNL001 plasmid. The inducer anhydrotetracycline (aTc), which binds to the tet repressor, controls the expression level of YFP-fused-T7 RNAP. Then, the genes encoding CFP and mCherry, which are integrated into E. coli genomic DNA, are expressed by T7 RNAP. Two Lac operators (O1) are located upstream and downstream of the T7 promoter. To achieve full expression of CFP and mCherry, 1 mM isopropyl β- D -1-thiogalactopyranoside (IPTG) was added. ( b ) Representative phase contrast, YFP, CFP and mCherry images of E. coli NL010 carrying pNL001. Scale bar, 10 μm. ( c ) Steady-state distributions of YFP-T7 RNAP at different aTc concentrations. Each distribution fits a gamma distribution well (solid curves). ( d ) Correlation between the CFP and mCherry intensity in the NL010 strain, in which T7 RNAP is induced under an aTc concentration of 0.05 ng ml −1 (green curve in Fig. 1c ). Each point represents a cell, for which fluorescence intensities are normalized by the average intensities of the cell population. The distributions of the CFP (top) and mCherry (right) intensities are described well by the gamma functions (solid curves). Full size image CFP and mCherry expression via T7 RNAP in E. coli Intrinsic and extrinsic noise is typically measured based on the pairwise correlation between two fluorescent reporters [1] , [18] . Because RNAP is an essential protein, variation in RNAP concentration will alter cell growth conditions and metabolism significantly, thus investigation of RNAP-dependent effects on noise is challenging. To avoid such undesirable changes in growth conditions due to variation in RNAP concentrations, we used T7 RNAP instead of endogenous E. coli RNAP ( Fig. 1a ). We incorporated the genes encoding CFP and mCherry into the E. coli chromosome under the control of the T7 RNAP promoter ( Fig. 1a ): we replaced galK with cfp and intC with the mCherry gene, as reported by Elowitz et al. [1] , to maintain identical copy numbers of both genes during the cell cycles ( Supplementary Fig. 1 ). T7 RNAP fused with YFP was expressed from a low-copy-number plasmid (pNL001), and its expression level was controlled by the concentration of the inducer anhydrotetracycline (aTc). After growing cells in M9 minimal medium with glucose, the relative concentrations of YFP-T7 RNAP, CFP and mCherry in individual cells were measured by fluorescence microscopy ( Fig. 1b ). The expression level of T7 RNAP was effectively controlled by the aTc concentration, and the observed T7 RNAP distributions fit gamma distributions well ( Fig. 1c ) [22] . The intrinsic and extrinsic noise of each protein’s expression level was calculated based on pairwise correlations between the concentrations of CFP and mCherry ( Fig. 1d ) [1] . 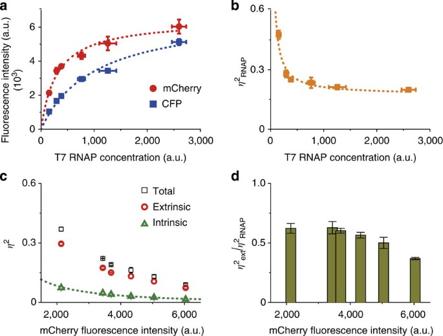Figure 2: Quantification of T7 RNAP noise and the intrinsic and extrinsic noises of downstream proteins. (a) Expression levels of CFP and mCherry by T7 RNAP at various aTc concentrations. (b) T7 RNAP noise obtained from the distribution of the YFP fluorescence intensity (Fig. 1c) as a function of the mean T7 RNAP concentration. The dotted line is fitted to the functiona/R+b1,15, whereR=the T7 RNAP concentration;a=38; andb=0.17. (c) The total (black open squares), extrinsic (red open circles) and intrinsic (green open triangles) noise of downstream protein expression, measured at each aTc concentration. Intrinsic noise is fitted to the functiona/P+b, whereP=mCherry fluorescence intensity;a=196; andb=−0.01 (dotted line). (d) The ratio of extrinsic noise to the RNAP noise, calculated at each aTc concentration. Error bars represent the mean±s.d. of three independent experiments. Figure 2a indicates that the expression levels of CFP and mCherry are dependent on T7 RNAP concentration: at high T7 RNAP concentrations, the expression levels of both proteins are close to saturation ( Fig. 2a ). Figure 2: Quantification of T7 RNAP noise and the intrinsic and extrinsic noises of downstream proteins. ( a ) Expression levels of CFP and mCherry by T7 RNAP at various aTc concentrations. ( b ) T7 RNAP noise obtained from the distribution of the YFP fluorescence intensity ( Fig. 1c ) as a function of the mean T7 RNAP concentration. The dotted line is fitted to the function a / R + b [1] , [15] , where R =the T7 RNAP concentration; a =38; and b =0.17. ( c ) The total (black open squares), extrinsic (red open circles) and intrinsic (green open triangles) noise of downstream protein expression, measured at each aTc concentration. Intrinsic noise is fitted to the function a / P + b , where P =mCherry fluorescence intensity; a =196; and b =−0.01 (dotted line). ( d ) The ratio of extrinsic noise to the RNAP noise, calculated at each aTc concentration. Error bars represent the mean±s.d. of three independent experiments. Full size image Quantifying the noise of downstream proteins From the distributions of RNAP concentrations ( Fig. 1c ), we measured noise in T7 RNAP under each inducer concentration ( Fig. 2b ). The noise was calculated based on variance over the squared mean of the T7 RNAP concentration in a population ( η 2 =( σ / μ ) 2 ). The noise in T7 RNAP ( ) converged to 0.2, which is relatively high compared with the noise of other proteins expressed from the E. coli genome [9] . Figure 2c shows the noise of downstream proteins at each inducer concentration. The intrinsic noise ( , green triangles) was inversely proportional to mCherry expression, which varied due to the different concentrations of T7 RNAP. This is consistent with previous work, in which protein expression level was modulated by different inducer concentrations [1] . The intrinsic noise was relatively low, contributing <20% of the total noise, and the majority of noise therefore came from extrinsic noise ( , red circles) in this gene-expression system. It is to be noted that the extrinsic noise of the downstream proteins was consistently lower than the noise in RNAP itself, regardless of protein expression level ( Fig. 2d ). This observation indicates that RNAP noise is not simply added or amplified to downstream protein noise, but attenuated by an unidentified factor. Thus, we further investigated how RNAP noise propagates to affect downstream protein levels [23] . To directly prove the propagation of RNAP noise to downstream proteins, one had to vary RNAP noise while a constant mean RNAP concentration was maintained. However, such conditions are not practically achievable using natural gene-expression systems due to the noise itself. We therefore investigated the mode of noise propagation by randomly generating cell distributions with pre-determined means and s.d. of the RNAP concentration from the total collection of cells ( Fig. 3a , left panel). We combined all of the cells generated under various aTc concentrations in Fig. 1c , and then randomly selected 500 cells from the total cell data (~40,000 cells) to obtain pre-determined means and s.d. of the RNAP concentration. To mimic the natural distribution of expression levels, we selected cells so that the resulting distribution of the T7 RNAP concentration in the subset of cells corresponded to a gamma distribution ( Fig. 3a , middle panel) [9] , [22] . Cells with similar concentrations of T7 RNAP expressed similar levels of CFP and mCherry, regardless of aTc induction conditions ( Supplementary Fig. 2 ). Using the selected subset of cells, we then calculated the RNAP noise and the intrinsic and extrinsic noises of downstream proteins ( Fig. 3a , middle and right panels). We repeated this process with fixed average RNAP concentrations while varying RNAP noise ( Fig. 3b–e ). 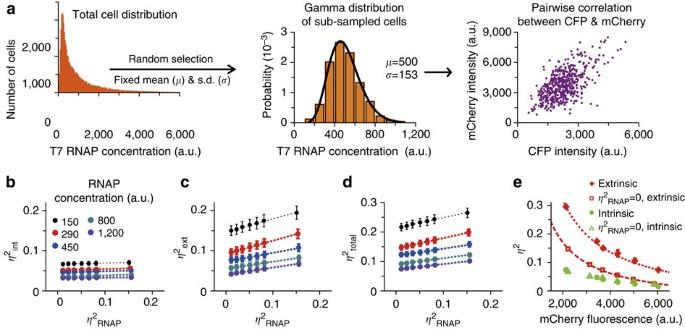Figure 3: Analysis of RNAP noise-dependent intrinsic and extrinsic noise. (a) Random generation of cell distributions with a pre-determined mean and s.d. of the RNAP concentration from the total collection of cells. Left, total cell distributions obtained by combining all cells fromFig. 1c(~40,000 cells). Middle, distribution of the subset of cells (500 cells) randomly selected from the total cell distribution to satisfy a given gamma distribution with a pre-determined mean (μ) and s.d. (σ). Right, pairwise correlation between the CFP and mCherry intensities in the sub-sampled cells. (b–d) Intrinsic, extrinsic and total noise of the sub-sampled cells depending on RNAP noise. The dotted lines represent linear guidelines for clarity. Error bars indicate±s.d.,n=1,000. (e) Contribution of RNAP noise to intrinsic and extrinsic noise. We compared the gene expression noises shown inFig. 2cwith those at an RNAP noise=0. The intrinsic and extrinsic noises at an RNAP noise=0 (open symbols) were obtained from theyaxis intercepts resulting from linear fitting inbandc, respectively. Figure 3: Analysis of RNAP noise-dependent intrinsic and extrinsic noise. ( a ) Random generation of cell distributions with a pre-determined mean and s.d. of the RNAP concentration from the total collection of cells. Left, total cell distributions obtained by combining all cells from Fig. 1c (~40,000 cells). Middle, distribution of the subset of cells (500 cells) randomly selected from the total cell distribution to satisfy a given gamma distribution with a pre-determined mean ( μ ) and s.d. ( σ ). Right, pairwise correlation between the CFP and mCherry intensities in the sub-sampled cells. ( b – d ) Intrinsic, extrinsic and total noise of the sub-sampled cells depending on RNAP noise. The dotted lines represent linear guidelines for clarity. Error bars indicate±s.d., n =1,000. ( e ) Contribution of RNAP noise to intrinsic and extrinsic noise. We compared the gene expression noises shown in Fig. 2c with those at an RNAP noise=0. The intrinsic and extrinsic noises at an RNAP noise=0 (open symbols) were obtained from the y axis intercepts resulting from linear fitting in b and c , respectively. Full size image Figure 3b demonstrates that the intrinsic noise of downstream proteins was nearly invariant with respect to RNAP noise. However, extrinsic noise increased with an increase in RNAP noise ( Fig. 3c ), and as a consequence, the total noise increased linearly ( Fig. 3d ). Figure 3e shows the contribution of RNAP noise to intrinsic and extrinsic noise: although removing RNAP noise had a negligible effect on intrinsic noise, extrinsic noise was significantly reduced. These results clearly demonstrate the long-lasting prediction that RNAP concentration variation, one of the global factors involved in gene expression, contributes to extrinsic, but not intrinsic noise [1] , [2] , [15] , [16] . Real-time analysis of the single-cell lineage Because we measured the concentration of RNAP at a given time point for the noise analysis, the history of the fluctuation in RNAP concentration was not fully considered in our sampling approach [24] , [25] . For example, although the RNAP concentration may be identical in two cells at the sampling point, the expression levels of the downstream proteins could differ in these two cells depending on the fluctuation history of the RNAP concentration of each cell. In this case, selecting a subset of cells to have a specific amount of RNAP noise does not guarantee that the noise of the downstream proteins of the selected cells includes the effect of the pre-determined amount of RNAP noise that we chose during the selection step. However, for less marked fluctuations of RNAP concentration, the RNAP concentration at a given time maintains much of the correlation with the concentrations of downstream proteins; thus, our sampling approach can reduce or increase the contribution of RNAP concentration noise on the extrinsic noise of downstream proteins. We measured the real-time fluctuation in RNAP concentration by monitoring its concentration at the single-cell level using a gel pad ( Supplementary Fig. 3 ; Supplementary Movie 1 ). The concentration of T7 RNAP increased with the addition of the inducer, aTc, and then reached a steady-state condition after ~2 h of induction ( Fig. 4a ). The concentrations of T7 RNAP at the steady state presented considerable heterogeneity within the cell population ( Fig. 4b ), but the T7 RNAP concentrations of most cells remained at the steady-state level for 3 h after reaching the steady state. The s.d. of the normalized T7 RNAP concentration at the steady state was ~10% for 2 h ( Fig. 4c ); that is, the T7 RNAP concentration fluctuated <20% (2 σ ) with a 95% confidence interval. In line with this real-time measurement of T7 RNAP fluctuation, the correlation coefficient ( r ) between the RNAP concentration and the concentrations of the downstream proteins of the cells used for the analysis in Fig. 3 was measured to be 0.88 for CFP and 0.74 for mCherry from the joint-probability distributions between the RNAP concentration and CFP and mCherry concentrations, respectively ( Supplementary Fig. 4 ). This result shows that RNAP concentration does not fluctuate to an extent that significantly disrupts the correlation between RNAP and its downstream proteins at the sampling time. 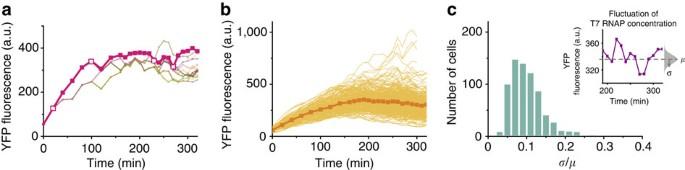Figure 4: Real-time observation of fluctuation in T7 RNAP concentration. (a) Time traces of YFP-T7 RNAP fluorescence intensity in single-cell lineages. The pink bold line follows a single lineage, and the other daughter cells have different light-coloured lines. Each open rectangle indicates cell division. (b) All time traces of T7 RNAP concentration (total 792 traces). The bold orange line represents the average intensity of YFP-T7 RNAP. (c) Analysis of the fluctuation in T7 RNAP concentration. After a steady-state condition was reached, we obtained the mean (μ) and s.d. (σ) of T7 RNAP intensity from 2 h of each time trace (inset). The histogram shows the s.d. of T7 RNAP intensity relative to the mean T7 RNAP intensity in a single time trace. The average relative s.d. (σ/μ) of T7 RNAP intensity in the time traces is 10±4%. Figure 4: Real-time observation of fluctuation in T7 RNAP concentration. ( a ) Time traces of YFP-T7 RNAP fluorescence intensity in single-cell lineages. The pink bold line follows a single lineage, and the other daughter cells have different light-coloured lines. Each open rectangle indicates cell division. ( b ) All time traces of T7 RNAP concentration (total 792 traces). The bold orange line represents the average intensity of YFP-T7 RNAP. ( c ) Analysis of the fluctuation in T7 RNAP concentration. After a steady-state condition was reached, we obtained the mean ( μ ) and s.d. ( σ ) of T7 RNAP intensity from 2 h of each time trace (inset). The histogram shows the s.d. of T7 RNAP intensity relative to the mean T7 RNAP intensity in a single time trace. The average relative s.d. ( σ / μ ) of T7 RNAP intensity in the time traces is 10±4%. Full size image This result may also explain the observation that the intrinsic noise of downstream proteins is invariant under changes in the magnitude of the T7 RNAP concentration noise [20] . Because temporal fluctuations in T7 RNAP abundance remain small relative to variation in RNAP abundance between cells for extended time intervals, the autocorrelation lifetime of RNAP fluctuation is much longer than the average lifetime of intrinsic fluctuations of the downstream protein, and the adjustment of downstream protein gene expression to changes in RNAP concentration is effectively instantaneous. Therefore, the possible contribution by dynamic fluctuation of RNAP concentration [24] to intrinsic noise in downstream gene expression, as measured by a dual reporter system, could be negligible under changes in the magnitude of T7 RNAP expression noise when the mean of the T7 RNAP concentration is held constant. Next, to quantitatively investigate the effect of the T7 RNAP concentration history on downstream noise, we measured the concentrations of the downstream proteins together with T7 RNAP concentration at the single-cell level on a gel pad for~5 h ( Fig. 5a,b ). We observed that CFP and mCherry concentrations reached a steady state after ~3 and 4.5 h of induction, respectively. The difference in expression curve may originate from the difference between the maturation times of CFP and mCherry. To evaluate the effect of the previous T7 RNAP expression levels on downstream protein noises, we integrated the fluorescence intensity of T7 RNAP in each cell lineage for 0 min (no integration), 30 min, 1 h and 2 h (~1.4 cell cycles on a gel pad) prior to the reference point (320 min) ( Fig. 5c ). Integrating T7 RNAP intensity for a specific period of time would account for the history of the RNAP concentration fluctuation. Next, we used the integrated fluorescence intensities of T7 RNAP for the random cell selection with fixed mean and variance as in Fig. 3a . We used the CFP and mCherry concentrations of the selected cells measured at 320 min for downstream noise analysis ( Fig. 5d–f ) (see Methods for a detailed description). We also tested CFP and mCherry concentrations at time points other than 320 min for the noise analysis in a similar manner ( Supplementary Fig. 5 ). In all cases, we found that the magnitudes of intrinsic and extrinsic noise of the downstream proteins were nearly independent of the integration time of T7 RNAP concentration within the error bar, indicating that fluctuation of T7 RNAP is not significant. Importantly, the intrinsic noise was invariant to RNAP noise variation, while extrinsic noise was linearly proportional to the RNAP noise in the gel-pad experiment. These results are in line with the results in Fig. 3 , which were obtained from cells grown in a shaking culture. These results consistently support our observation that RNAP concentration variation contributes mostly to extrinsic noise. In addition, selecting cells with particular RNAP concentrations is a valid approach for controlling extrinsic perturbation by RNAP in our gene-expression system, because the fluctuation history of the T7 RNAP concentration presented a minimal effect on downstream protein noises. 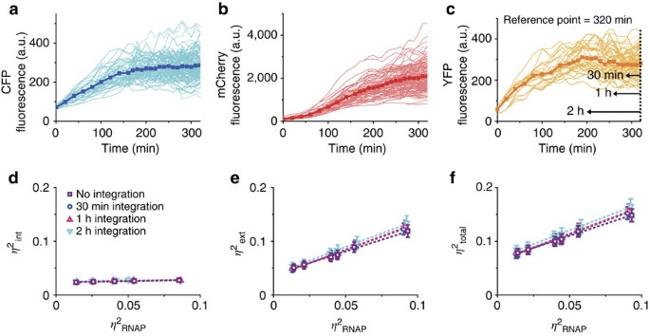Figure 5: Evaluation of the effect of the T7 RNAP concentration history on downstream protein noise at the single-cell lineage level. Together with T7 RNAP intensity, the intensities of CFP and mCherry were measured for ~5 h. We used 729 traces for the analysis but showed only 200 traces ina–cfor clarity. Representative time traces of (a) CFP fluorescence intensity and (b) mCherry fluorescence intensity. The bold blue and red lines indicate the average. (c) Representative time traces of YFP-T7 RNAP fluorescence intensity. The integration times for YFP-T7 RNAP concentration of a single-cell lineage, 0, 30, 1 and 2 h from the reference point (320 min), are indicated. (d–f) Dependence of the intrinsic, extrinsic and total noise of the sub-sampled cells on RNAP noise. Here, we used the integrated YFP-T7 RNAP concentrations fromFig. 5cfor the subsampling analysis, and the concentrations of CFP and mCherry of the selected cells measured at 320 min were used for noise analysis in a population. The dotted lines represent linear guidelines for clarity. Error bars indicate±s.d.,n=1,000. Figure 5: Evaluation of the effect of the T7 RNAP concentration history on downstream protein noise at the single-cell lineage level. Together with T7 RNAP intensity, the intensities of CFP and mCherry were measured for ~5 h. We used 729 traces for the analysis but showed only 200 traces in a – c for clarity. Representative time traces of ( a ) CFP fluorescence intensity and ( b ) mCherry fluorescence intensity. The bold blue and red lines indicate the average. ( c ) Representative time traces of YFP-T7 RNAP fluorescence intensity. The integration times for YFP-T7 RNAP concentration of a single-cell lineage, 0, 30, 1 and 2 h from the reference point (320 min), are indicated. ( d – f ) Dependence of the intrinsic, extrinsic and total noise of the sub-sampled cells on RNAP noise. Here, we used the integrated YFP-T7 RNAP concentrations from Fig. 5c for the subsampling analysis, and the concentrations of CFP and mCherry of the selected cells measured at 320 min were used for noise analysis in a population. The dotted lines represent linear guidelines for clarity. Error bars indicate±s.d., n =1,000. Full size image Calculating the dependence of downstream protein noises on RNAP noise from a single-cell lineage at the steady-state RNAP concentration is an alternative way of investigating RNAP noise effect ( Supplementary Fig. 6 ). However, RNAP noise in a single-cell lineage at the steady state was extremely low ( Fig. 4c ) and thus it was difficult to observe any dependence of protein noise on RNAP noise ( Supplementary Fig. 6a–c ). The noise of RNAP measured from a single-cell lineage ( Fig. 4c ) was smaller than the noise from a cell population. This difference occurred because the observation duration for a single-cell lineage was not long enough to satisfy ergodicity, consistent with other works [9] , [15] . Thus, a subsampling approach is required in this study. Then, because the real-time tracking data in Fig. 5a–c reported variation in RNAP concentration as well as that of the downstream protein concentrations of each single-cell lineage, we calculated RNAP noise and intrinsic, extrinsic and total noise of the downstream proteins of each single-cell lineage using concentration data from the induction point (0 min) to 320 min (total 729 cells) ( Supplementary Fig. 6d–f ). This noise includes the variation in the RNAP concentration caused by induction; thus, this noise is not the same as traditionally defined noise, which is typically obtained at steady state. However, this noise can be used to approximate the large dynamic effects of RNAP concentration fluctuation. Interestingly, intrinsic noise was nearly independent of RNAP noise, while extrinsic noise increased linearly as the RNAP noise of each cell lineage increased ( Supplementary Fig. 6g ); this result further supports our finding that RNAP noise propagates to the extrinsic noise of the downstream proteins. Model of RNAP noise propagation We note that the dependency of extrinsic noise on RNAP noise (slope in Fig. 3c ) decreased as the expression level of T7 RNAP was increased: the magnitude of the slope determines the ‘propagation efficiency’ of RNAP noise to downstream proteins. This observation indicated that the propagation of RNAP noise was dependent on T7 RNAP concentration. As RNAP concentration was increased, the extent of the propagation of RNAP noise was reduced. To assess what determines the propagation efficiency of RNAP noise, we considered the kinetic scheme of transcription given by the following description: where k 1 and k − 1 are the rate coefficients for the association and dissociation reactions between RNAP and the promoter, respectively, and k 2 is the transcriptional initiation rate for mRNA synthesis. According to Michaelis–Menten enzyme kinetics, the steady-state rate of the above transcriptional reaction is proportional to θ = KN RNAP /(1+ KN RNAP ), where K is defined by K = k 1 /( k 2 + k −1 ) and N RNAP is the RNAP concentration. Here, θ and K can be interpreted as the fraction of the promoter occupied by RNAP during the transcriptional reaction and the affinity of RNAP for the promoter, respectively. Then, the overall transcriptional rate ( R TX ) can be defined as R TX = k TX θ (0< θ <1), where k TX denotes the overall transcriptional rate when θ is unity. By definition, k TX is independent of RNAP concentration. In contrast, the fraction of RNAP occupation (or the unoccupied fraction, 1− θ ) is dependent on RNAP concentration. Thus, only the fraction of promoter occupation by T7 RNAP is a potential factor responsible for the propagation of RNAP noise in this kinetic scheme. If the fraction of occupation becomes unity (or the unoccupied fraction becomes zero), fluctuations in RNAP concentration would have no effect on the variation of transcription and protein expression. Thus, if the fraction of occupation is related to noise propagation, the slope, or the propagation efficiency of RNAP noise as shown in Fig. 3c , should converge to zero as the RNAP concentration reaches a saturation level, that is, when the fraction of occupation is close to unity. To test this hypothesis, we prepared a high-copy-number plasmid (pNL002) to express T7 RNAP at sufficiently high levels to saturate the expression levels of both CFP and mCherry ( Supplementary Fig. 7 ). We performed the same random selection procedure for subsets of cells to achieve a gamma distribution as indicated in Fig. 3a ( Supplementary Fig. 8 ) and quantified intrinsic and extrinsic noise values depending on RNAP noise at constant RNAP concentrations ( Fig. 6a–c ). Consistent with our prediction, extrinsic and intrinsic noise were nearly invariant with respect to variation in RNAP noise (slope<0.03) ( Fig. 6b ); that is, the propagation efficiency of RNAP noise was close to zero. As a consequence, the total noise was also invariant with respect to the RNAP noise ( Fig. 6c ). We found that the propagation efficiencies obtained from the extrinsic noise well fit the function of the unoccupied fraction, (1− θ )= a /(1+ KN RNAP ) ( Fig. 6d ). These results demonstrated that the propagation of RNAP noise to downstream protein noise depends on the RNAP concentration. We propose that the fraction of occupation of the promoter determines the efficiency of noise propagation. For a given distribution of RNAP concentrations, a gene with a stronger promoter is less susceptible to RNAP noise, thus propagating RNAP noise to downstream protein expression less efficiently. 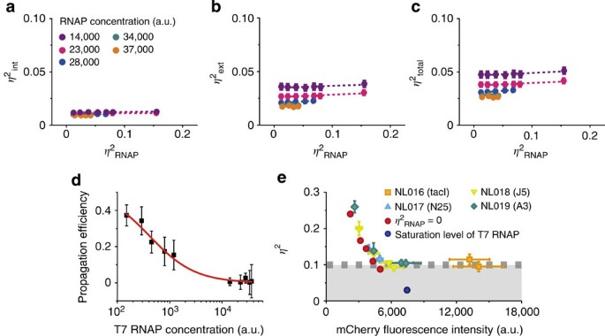Figure 6: Analysis of RNAP-dependent intrinsic and extrinsic noise at saturation conditions. (a) Intrinsic, (b) extrinsic and (c) total noises of the sub-sampled cells depending on RNAP noise using the high-copy-number plasmid (pNL002). We expressed T7 RNAP at a sufficiently high level using pNL002 to saturate the expression levels of CFP and mCherry (Supplementary Fig. 7), and generated sub-sampled cell distributions of RNAP concentrations with pre-determined means and s.d. from the total collection of cells (Supplementary Fig. 8). The dotted lines represent linear guidelines for clarity. Error bars indicate±s.d.,n=1,000. (d) The slope (susceptibility to RNAP noise) of the extrinsic noise depending on the T7 RNAP concentration fromFigs 3cand6b. The red line is fitted to the function of the unoccupied fraction of the promoter by RNAP,a/(1+KR), whereRandKdenote T7 RNAP concentration and the RNAP affinity for the promoter, respectively (least squares,R2=0.99). Error bars indicate±s.d.,n=10. (e) Comparison of mCherry noise induced by variousE. coliRNAP promoters with the noise induced by T7 RNAP promoters. The rectangle, triangle and diamond symbols represent the gene expression noise under variousE. coliRNAP promoters20. Expression levels in each strain were modulated by applying different IPTG concentrations. When mean mCherry intensity is >6,000 (a.u.), noise becomes saturated at ~0.1 (dashed line), consistent with the findings of Taniguchiet al.9Error bars represent the mean±s.d. of three independent experiments. The red-filled circles represent gene expression noise under the T7 promoter when the noise induced by the RNAP noise is removed, as estimated from the linear fitting shown inFig. 3c. The blue-filled circle represents gene expression noise under the T7 promoter at saturation-level T7 RNAP concentrations using pNL002. Figure 6: Analysis of RNAP-dependent intrinsic and extrinsic noise at saturation conditions. ( a ) Intrinsic, ( b ) extrinsic and ( c ) total noises of the sub-sampled cells depending on RNAP noise using the high-copy-number plasmid (pNL002). We expressed T7 RNAP at a sufficiently high level using pNL002 to saturate the expression levels of CFP and mCherry ( Supplementary Fig. 7 ), and generated sub-sampled cell distributions of RNAP concentrations with pre-determined means and s.d. from the total collection of cells ( Supplementary Fig. 8 ). The dotted lines represent linear guidelines for clarity. Error bars indicate±s.d., n =1,000. ( d ) The slope (susceptibility to RNAP noise) of the extrinsic noise depending on the T7 RNAP concentration from Figs 3c and 6b . The red line is fitted to the function of the unoccupied fraction of the promoter by RNAP, a /(1+ KR ), where R and K denote T7 RNAP concentration and the RNAP affinity for the promoter, respectively (least squares, R 2 =0.99). Error bars indicate±s.d., n =10. ( e ) Comparison of mCherry noise induced by various E. coli RNAP promoters with the noise induced by T7 RNAP promoters. The rectangle, triangle and diamond symbols represent the gene expression noise under various E. coli RNAP promoters [20] . Expression levels in each strain were modulated by applying different IPTG concentrations. When mean mCherry intensity is >6,000 (a.u. ), noise becomes saturated at ~0.1 (dashed line), consistent with the findings of Taniguchi et al. [9] Error bars represent the mean±s.d. of three independent experiments. The red-filled circles represent gene expression noise under the T7 promoter when the noise induced by the RNAP noise is removed, as estimated from the linear fitting shown in Fig. 3c . The blue-filled circle represents gene expression noise under the T7 promoter at saturation-level T7 RNAP concentrations using pNL002. Full size image Dominant source of the extrinsic noise in E. coli Recently, Taniguchi et al. [9] reported that the noise associated with bacterial proteins converged to a limit of 0.1 when they measured the noises of nearly 1,000 E. coli proteins. This noise limit, generally attributed to residual extrinsic noise [1] , [9] , [13] , [26] , has also been observed in yeast [12] . Because the noise measured by counting mRNA copy numbers is mostly intrinsic [21] , [27] , translational noise or the noise generated by other metabolites is attributed to the source of this extrinsic noise limit [18] . We tested whether the extrinsic noise limit was retained when the portion of extrinsic noise induced by RNAP noise was minimized. We first tested whether the extrinsic noise limit expressed by endogenous E. coli RNAP was observed under our noise-measurement conditions. We incorporated the mCherry gene into the E. coli chromosome under various E. coli RNAP promoters and then measured the total noise. As expected, the noise reached a saturation floor at 0.1 for cells grown in M9 glucose minimal medium ( Fig. 6e ), consistent with the findings of Taniguchi et al. [9] However, when saturating levels of T7 RNAP were induced using pNL002 to minimize the noise caused by RNAP fluctuations ( Fig. 6c ), the total noise was reduced to 0.03 ( Fig. 6e , blue-filled circles). This result demonstrates that the noise generated by ribosomes and translational fluctuation, as well as the fluctuation of other metabolisms can be as low as 0.03 in E. coli . The red-filled circles in Fig. 6e represent the total noise observed after subtracting RNAP noise-induced extrinsic noise, which was consistently smaller than the noise of E. coli RNAP-driven expression at identical mCherry expression levels. Because the translation process in our bacterial system is identical to that of natural E. coli , the reduction of the minimum noise from 0.1 in natural E. coli to 0.03 in our cell system can be mostly ascribed to replacement of the bacterial transcription system with the viral system. A total of 70% of the minimum noise is a result of fluctuation in the transcriptional process of highly expressed genes in E. coli , whereas the noise resulting from translational fluctuation is <30% of the minimum gene expression noise in natural E. coli genes. Transcriptional bursting, the origin of which is still unknown in bacteria [21] , [27] , transcription factor dynamics [28] , transcriptional pausing or the complicated process of E. coli RNAP initiation with sigma factor binding, such as open complex formation and abortive initiation [29] , [30] , may contribute to the transcriptional noise of E. coli RNAP. Another possible mechanism for generating such noise is transient variation in the concentration of E. coli RNAP available for the specific promoter due to intensive RNAP use by other promoters. Generally, bacteria and higher organisms display high-copy-number RNAPs. However, they also exhibit high copy numbers of promoters for RNAP binding, and thus the available number of RNAPs near a specific promoter may transiently fluctuate. Our results indicate that such local effects, if present, should be transmitted to downstream protein expression noise. The probability of promoter occupation by RNAP may determine what fraction of RNAP noise is transmitted to downstream protein noise. In summary, we have demonstrated that RNAP noise is transmitted to downstream protein noise as an extrinsic noise factor ( Supplementary Fig. 9 ). The propagation of RNAP noise to downstream protein noise was attenuated and is inversely proportional to RNAP concentration. When the downstream noise induced by RNAP noise was removed by saturating promoter occupancy, the total noise was reduced to 30% of the lower limit of the noise in E. coli , suggesting that noise generated at the transcriptional level is the dominant source of the extrinsic noise of high-copy-number proteins in bacteria. pNL001 and pNL002 plasmids for T7 RNAP expression T7 RNAP fused with YFP ( Venus ) [31] was expressed from a low-copy-number plasmid (pNL001), which was tightly regulated by the tet promoter and carried the ampicillin-resistant gene ( ampR ). The expression of T7 RNAP was induced by anhydrotetracycline (aTc). When a saturation level of T7 RNAP was required, YFP-fused T7 RNAP was expressed from a high-copy-number plasmid (pNL002). L -arabinose was used to induce T7 RNAP expression from pNL002, which also carries ampR for antibiotic selection. NL010 strain We constructed an E. coli strain (NL010) expressing CFP and mCherry via T7 RNAP. We replaced intC with the mCherry gene and galK with cfp (the CFP gene) in the E. coli chromosome using λ-RED recombination. The inserted region included two lac operators (O1), a T7 promoter, a ribosome-binding site, a gene encoding a fluorescent protein and the cat (chloramphenicol resistance) gene ( Fig. 1a ). We inserted two O1 sequences both upstream and downstream of the T7 promoter to reduce the background level of protein expression. The cat gene was removed using a FRT cassette following successful insertion of the target gene into genomic DNA. NL016—NL019 strains To test the lower noise limit in E. coli , we inserted the mCherry gene under various E. coli RNAP promoters. The promoter sequences employed are referred to in the literature [32] . The inserted sequences included a promoter, O1, ribosome-binding site, the mCherry gene and cat . We replaced the lac operon with these sequences using λ-RED recombination. (promoter sequences: from −50 to +1) NL016 (PtacI): 5′-ttctgaaatgagctgttgacaattaatcatcggctcgtataatgtgtgga-3′ NL017 (PN25): 5′-tcataaaaaatttatttgccttcaggaaaatttttctgtataatagattca-3′ NL018 (PJ5): 5′-atataaaaaccgttattgacacaggtggaaatttagaatatactgttagta-3′ NL019 (PA3): 5′-ggtgaaacaaaacggttgacaacatgaagtaaacacggtacgatgtaccaca-3′ Cell preparation All strains were grown overnight in LB medium at 37 °C from a single colony. The overnight cultures were re-inoculated into fresh M9 medium supplemented with 0.4% glucose, amino acids and vitamins at 1:200 dilution, unless otherwise specified. The cells were grown at 37 °C until reaching an OD 600 ~0.3, and a 1-ml aliquot of the cells was then pelleted by centrifugation for 1 min and resuspended in 500 μl of fresh M9 medium for washing. The cells were pelleted again by centrifugation and resuspended in a final volume of 5 μl fresh M9 medium. Then, 0.8 μl of the concentrated cell culture was placed between a coverslip and a 3% low-melting-temperature agarose gel pad (Lonza, #50111) prepared with M9 medium. NL010 cells carrying the pNL001 plasmid were induced with aTc at final concentrations of 0, 0.01, 0.02, 0.05, 0.1 and 1 ng ml −1 to modulate the expression level of T7 RNAP. To achieve full expression of CFP and mCherry, 1 mM isopropyl β- D -1-thiogalactopyranoside (IPTG) was added together with aTc. For the NL010 carrying the pNL002 plasmid, M9 medium supplemented with 0.4% glycerol was used to achieve a high expression level of the pNL002 plasmid, together with 0.1 and 0.2% of L-arabinose. Microscope setup Samples were placed on an inverted microscope (Olympus, IX-71) with a × 100 oil-immersed objective lens (Olympus). Phase contrast images and three fluorescence images for CFP, YFP and mCherry were acquired at multiple positions using a cooled EMCCD camera (Andor iXon DU897). For CFP, FF01-434/17-25 (excitation), FF01-479/40-25 (emission) and FF452-Di01-25 × 36 (dichroic mirror) were used (purchased from Semrock). For mCherry, FF01-572/28-25 (excitation), FF01-641/75-25 (emission) and FF593-Di02-25 × 36 (dichroic mirror) were used. For YFP, FF01-500/24-25 (excitation), FF01-550/32-25 (emission) and Q525LP (dichroic mirror) were used. Metamorph software (Molecular Devices) was employed to control the automated measurements and maintain focus during data acquisition. Image analysis The images were analysed using home-built software (Matlab). The program extracted the total fluorescence intensity of individual cells from the phase contrast and fluorescence images automatically and recorded the average fluorescence intensity (concentration) by normalizing the total intensity to the cell area. The intensity of autofluorescence was obtained from NL010 cells without the plasmid expressing YFP-T7 RNAP. Noise analysis by generating gamma distributions We generated gamma distributions based on the YFP fluorescence intensities in cells to obtain pre-determined means ( μ ) and s.d. ( σ ). We prepared the total cell collection by combining all cells obtained from the measurements performed at different aTc concentrations ( Fig. 3a ). The number of cells in the entire collection was ~40,000. Then we randomly selected 500 cells each time from the total cell collection to satisfy a given gamma distribution: with a = μ 2 / σ 2 and b = σ 2 / μ being fixed, following the procedure described below. 1 Using input values for the mean ( μ ) and s.d. ( σ ), we calculated a = μ 2 / σ 2 and b = σ 2 / μ and obtained the gamma distribution, . 2 We set the size of the bin for the X-axis (YFP intensity) to σ /2. Then, we calculated the number of cells required for each bin to satisfy the given gamma distribution. We set the total number of the sub-sampled cells as 500. 3 We randomly selected the required number of the cells for each bin from the total cell collection. 4 The selected cells were used to calculate the intrinsic, extrinsic and total noises as follows, as defined by Elowitz et al. [1] : where c and m represent the CFP and mCherry fluorescence intensity in each cell, respectively. 5 The mean and s.d. of the noises were obtained by repeating this process of random selection 1,000 times. Real-time observation of single-cell lineage on a gel pad For real-time experiments, NL010 cells carrying the pNL001 plasmid were grown in LB overnight. The overnight cultures were re-inoculated into fresh M9 medium supplemented with 0.4% glucose, amino acids and vitamins at 1:200 dilution. For maintenance of the basal expression level of CFP and mCherry, the cells were grown in the presence of 1 mM IPTG at 37 °C until they reached ~0.2 OD 600 . Then, a 500-μl aliquot of the cells was pelleted by centrifugation and resuspended in a final volume of 50 μl of fresh M9 medium, and 0.5 μl of the cells was placed between a coverslip and a 1.5% low-melting-temperature agarose gel pad (Lonza, #50111) prepared with M9 media containing 1 ng ml −1 aTc and 1 mM IPTG. The sample chamber was attached to a temperature controller (FCS2, Bioptechs) and maintained at 37 °C during the experiments. To provide a continuous flow of fresh media, pre-warmed M9 media containing 1 ng ml −1 aTc and 1 mM IPTG was supplied by a syringe pump at 0.26 ml min −1 . Images were acquired every 20 min for 160 min and then every 10 min for the remaining time. The acquired images were analysed using the Schnitzcell MATLAB module (provided by the M. Elowitz group, California Institute of Technology) [33] . Analysis of the T7 RNAP history effect on the protein noise To quantitatively investigate the effect of the T7 RNAP concentration history, we integrated YFP-T7 RNAP intensities for each cell lineage for a specific period of time (0, 30, 1 and 2 h) from the reference time point (320 min), as depicted in Fig. 5c . Then, we used the integrated YFP-T7 RNAP intensity of each cell for random cell selection with a fixed mean and variance, similar to our selection in Fig. 3a . We randomly selected 300 cells each time from the 729 total cells to satisfy a given gamma distribution: with a = μ 2 / σ 2 and b = σ 2 / μ being fixed, and x =the integrated YFP-T7 RNAP intensity. The downstream protein noise was calculated using CFP and mCherry fluorescence intensities from measurements of the selected cells at the reference time point (320 min). We used the subsampling procedure described in ‘noise analysis by generating gamma distributions’ for the remaining procedure of the subsampling noise analysis. The mean and s.d. of the noise were obtained by repeating this process of random selection 1,000 times ( Fig. 5d–f ). How to cite this article: Yang, S. et al. Contribution of RNA polymerase concentration variation to protein expression noise. Nat. Commun. 5:4761 doi: 10.1038/ncomms5761 (2014).